A 150-million-year-old crab larva and its implications for the early rise of brachyuran crabs True crabs (Brachyura) are the most successful group of decapod crustaceans. This success is most likely coupled to their life history, including two specialised larval forms, zoea and megalopa. The group is comparably young, starting to diversify only about 100 million years ago (mya), with a dramatic increase in species richness beginning approximately 50 mya. Early evolution of crabs is still very incompletely known. Here, we report a fossil crab larva, 150 mya, documented with up-to-date imaging techniques. It is only the second find of any fossil crab larva, but the first complete one, the first megalopa, and the oldest one (other fossil ca. 110 mya). Despite its age, the new fossil possesses a very modern morphology, being indistinguishable from many extant crab larvae. Hence, modern morphologies must have been present significantly earlier than formerly anticipated. We briefly discuss the impact of this find on our understanding of early crab evolution. Among decapod crustaceans, true crabs (Brachyura) are by far the most successful evolutionary lineage. With approximately 7,000 extant species [1] , [2] , they represent the most species-rich distinct decapod morphotype [3] . Crabs furthermore have conquered nearly all habitats and numerous ecological niches. Most extant species are marine, but some 1,300 species are known from freshwater habitats [4] , and some species spend most of their life on dry land [5] . This species richness and ecological diversity is even more astonishing when considering the age of this group. The first representatives of Brachyura appear comparably late in the fossil record, in the Jurassic (about 180 mya), and start to diversify in the middle Cretaceous (about 100 mya) with a later increase of species richness in the Eocene (about 50 mya) [6] , [7] . Despite this somewhat late origin (as compared to other groups of decapod crustaceans), brachyuran crabs diversified extremely rapidly both morphologically and ecologically. Insights into the early evolution of crabs are hampered by two difficulties: (1) the true identity of their earliest representatives is a subject of debate [8] , [9] , and (2) early crab fossils are usually exclusively remains of the carapace [10] and thus of limited value in understanding the biology of these early forms. It is especially surprising that fossils of true crabs from the lithographic limestones of southern Germany, which are famous for their exceptional preservation of representatives of various decapod groups, are rare and usually of poor quality [11] ( Fig. 1a–f ), while crabs are well known and more common in other contemporary limestones [12] . 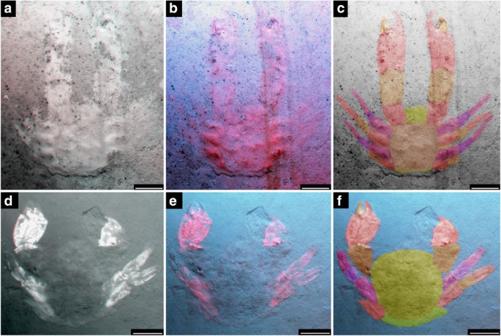Figure 1: Examples of adult brachyuran crabs or crab-like decapods, from the Solnhofen Lithographic Limestones. (a–c) Specimen A, collection Frattigiani, Laichingen (figured in ref.11). (d–f) Specimen B, collection Frattigiani, Laichingen. (a,d) Red-cyan stereo-anaglyphs, based on physical stereo-pairs. (b,e) Macrofluorescence images. (c,f) Colour-marked interpretations. Scale bars: 3 mm. Figure 1: Examples of adult brachyuran crabs or crab-like decapods, from the Solnhofen Lithographic Limestones. ( a – c ) Specimen A, collection Frattigiani, Laichingen (figured in ref. 11 ). ( d – f ) Specimen B, collection Frattigiani, Laichingen. ( a , d ) Red-cyan stereo-anaglyphs, based on physical stereo-pairs. ( b , e ) Macrofluorescence images. ( c , f ) Colour-marked interpretations. Scale bars: 3 mm. Full size image Part of the evolutionary success of brachyurans could be coupled to their life-history strategy, which usually involves a pronounced metamorphosis [13] , [14] . Most crabs develop through a few stages (usually 2 to as many as 8 or 9, depending on the group) of planktonic zoea larvae. The final zoea larva then moults into a still-swimming larva called a megalopa, which is morphologically and ecologically a transitional phase between the planktonic zoeae and the benthic adult [14] . The more general term ‘decapodid’ refers to this transitional larval phase in all of the Decapoda; the term ‘megalopa’ is most often used to denote the decapodid stage of true (brachyuran) crabs (but see ref. 15 ). The megalopa, after settling on an appropriate substrate, then moults into the first crab stage [14] . However, many deviations from this developmental sequence occur within Brachyura; certain larval phases can be skipped (usually called abbreviated development) [16] , and in some cases the hatchlings are already fully developed crabs (e.g., in most freshwater groups) [14] , a phenomenon often referred to as ‘direct development’ [14] , [16] . The developmental mode of early representatives of Brachyura is currently unknown. As demonstrated for other decapods, early representatives can have quite different developmental patterns compared to modern representatives [17] , [18] , [19] . To date, only a single occurrence of fossil crab larvae has been reported. That brief report was based on two rather fragmentary zoea specimens from the Cretaceous of Brazil. These incomplete fossils lacked appendages and a pleon, consisting only of the zoeal carapace and eye [20] , [21] . We report here a specimen from the Solnhofen Lithographic Limestones of southern Germany, about 150 mya. The fossil is remarkable in that it represents an exceptionally preserved brachyuran megalopa. It is thus only the second report of any fossilised crab larva, the first report of a well-preserved (nearly complete) fossil brachyuran larva, and the first record of a fossilised megalopa larva. We discuss the impact of this find in an evolutionary context. Taxonomic remarks Currently we cannot assign the specimen to a specific genus or species, nor can we definitely distinguish it from all other known (described) megalopa larvae of extant crab species. The reason for this is twofold: (1) the fossil megalopa, although preserved in surprising detail, does not provide enough characters to allow us to place it in any known group; and (2) megalopa larvae of extant species (where known) are often morphologically quite similar [14] , and there are very few keys to their identification. The modern appearance of the larva (its similarity to the megalopa larvae of several groups of extant crabs) suggests that it could belong to the higher crabs (Eubrachyura). However, even this is uncertain, as larval series for more ‘primitive’ crab groups (e.g., Dromiacea, Raninoida, Cyclodorrippoida, sometimes referred to as ‘podotreme’ crabs [2] , [22] ) are not well known. For reference the specimen is herein termed ‘Frattigiani’s megalopa’ in honour of the finder of the specimen, Roger Frattigiani, Laichingen, Germany. Description of the specimen Small sized immature decapod crustacean ( Figs 2a , 3a and 4a,d ). Shield formed by cephalothorax, round in outline, with a pronounced rostrum ( Figs 2e , 3c and 4b ); biforked spines flank the rostrum ( Figs 3c and 4b ). Marked cervical groove relatively far anterior ( Fig. 4d–f ); region anterior to cervical groove armed with numerous spines ( Figs 3c and 4b ). Anterior to rostrum small antennules with at least two articles, no flagella apparent. Second antenna with longer flagellum. Further posterior and laterally to the antennae are large bulbous structures, most likely representing the large, stalked eyes. Mouthparts unknown. Thoracopod 4 (pereopod 1) robust, carpus subtriangular, propodus about 2.5 times as long as wide ( Figs 2b and 3b ). Fixed finger of propodus and dactylus appear to form a chela, exact outlines unclear. Thoracopods 5–7 (8 partly unclear) more slender ( Fig. 3b ); consisting of seven articles; short articles 1–3 (coxa, basis, ischium), article 4 (merus) more elongate; articles 2–4 with numerous hook-like spines medially arranged in two rows ( Figs 2c and 3c ); article 5 (carpus) shorter; article 6 (propodus) elongate, slightly curved, also armed with spines, but smaller ones; article 7 (dactylus) elongate scimitar-shaped ( Fig. 2d ). Thoracopods arranged around sub-triangular sternum ( Fig. 4d–f ). Pleon with 6 segments ( Fig. 3d ); pleomere 1 trapezoidal in dorsal view; pleomere 2 wider and longer; pleomere 3 slightly wider, but shorter; pleomere 4 about as wide as 3, but shorter; pleomere 5 narrower, slightly longer; pleomere 6 narrower, significantly shorter; pleomeres 2–6 armed with numerous spines on their tergites ( Figs 2f , 3c and 4c ). Telson sub-triangular to sub-trapezoidal with two indistinct processes ( Fig. 3d ). 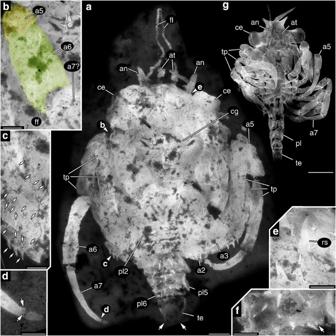Figure 2: New fossil brachyuran megalopa and modern megalopa for comparison. (a) Overview of Frattgiani’s megalopa (SMNS 70265) from the Solnhofen Lithographic Limestones, about 150 mya. (b) Color-marked close-up of thoracopod 4, cheliped, which is weakly compressed through the shield. (c) Close-up on proximal region of thoracopods 5–7; arrows mark the numerous spines. (d) Distal tip of a thoracopod (5–7); arrows mark small spines of about 8 μm in diameter. (e) Close-up on rostrum. (f) Close-up on spines of the pleomeres; arrow marks small spine. (g) Megalopa larva of the modern brachyuran crabHyas araneusin ventral view, for comparison. a, article; an, antenna; at, antennula; ce, compound eye; cg, cervical groove; ff, fixed finger; fl, flagellum; pl, pleomere; rs, rostrum; te, telson; tp, thoracopod. Scale bars: (a) 0.5 mm, (b) 300 μm, (c) 250 μm, (d–f) 200 μm, (g) 1 mm. Figure 2: New fossil brachyuran megalopa and modern megalopa for comparison. ( a ) Overview of Frattgiani’s megalopa (SMNS 70265) from the Solnhofen Lithographic Limestones, about 150 mya. ( b ) Color-marked close-up of thoracopod 4, cheliped, which is weakly compressed through the shield. ( c ) Close-up on proximal region of thoracopods 5–7; arrows mark the numerous spines. ( d ) Distal tip of a thoracopod (5–7); arrows mark small spines of about 8 μm in diameter. ( e ) Close-up on rostrum. ( f ) Close-up on spines of the pleomeres; arrow marks small spine. ( g ) Megalopa larva of the modern brachyuran crab Hyas araneus in ventral view, for comparison. a, article; an, antenna; at, antennula; ce, compound eye; cg, cervical groove; ff, fixed finger; fl, flagellum; pl, pleomere; rs, rostrum; te, telson; tp, thoracopod. Scale bars: ( a ) 0.5 mm, ( b ) 300 μm, ( c ) 250 μm, ( d – f ) 200 μm, ( g ) 1 mm. 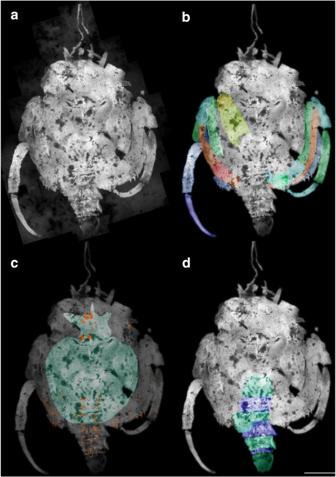Figure 3: Interpretation of dorsal and ventral structures of Frattigiani’s megalopa highlighted as colour markings. (a) Overview without markings of SMNS 70265. (b) Marking of appendages: thoracopod 4 (cheliped) in yellow; thoracopods 5–7 marked in green/cyan, orange/red and blue/indigo; exact identities difficult to judge; this interpretation is only an approximation. (c) Outline of shield (carapace) in green; all observed spines in orange. (d) Pleomeres in light green and blue and telson in darker green; pleon is in an anteriorly displaced position. Scale bar: 1 mm. Full size image Figure 3: Interpretation of dorsal and ventral structures of Frattigiani’s megalopa highlighted as colour markings. ( a ) Overview without markings of SMNS 70265. ( b ) Marking of appendages: thoracopod 4 (cheliped) in yellow; thoracopods 5–7 marked in green/cyan, orange/red and blue/indigo; exact identities difficult to judge; this interpretation is only an approximation. ( c ) Outline of shield (carapace) in green; all observed spines in orange. ( d ) Pleomeres in light green and blue and telson in darker green; pleon is in an anteriorly displaced position. Scale bar: 1 mm. 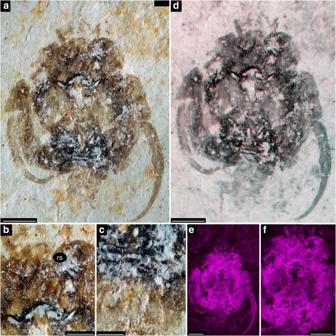Figure 4: Frattigani’s megalopa under different documentation methods. (a–c) Composite images under cross-polarised light. (a) Overview of SMNS 70265. (b) Close-up of rostrum; arrows mark biforked spines flanking the rostrum. (c) Close-up of spines on pleomeres. (d–f) Stereo images presented as red-cyan or red-blue anaglyphs (please use red-cyan glasses to view). (d) Physical stereo image. (e,f) Virtual surface reconstructions based on image stacks. (e) Overview. (f) Close-up on central body region. Ind–fthe stereo effect enhances especially the cervical groove, sternum, and leg insertions. rs, rostrum. Scale bars: (a,d–f) 1 mm, (b) 0.5 mm, (c) 0.3 mm. Full size image Figure 4: Frattigani’s megalopa under different documentation methods. ( a – c ) Composite images under cross-polarised light. ( a ) Overview of SMNS 70265. ( b ) Close-up of rostrum; arrows mark biforked spines flanking the rostrum. ( c ) Close-up of spines on pleomeres. ( d – f ) Stereo images presented as red-cyan or red-blue anaglyphs (please use red-cyan glasses to view). ( d ) Physical stereo image. ( e , f ) Virtual surface reconstructions based on image stacks. ( e ) Overview. ( f ) Close-up on central body region. In d – f the stereo effect enhances especially the cervical groove, sternum, and leg insertions. rs, rostrum. Scale bars: ( a , d – f ) 1 mm, ( b ) 0.5 mm, ( c ) 0.3 mm. Full size image Frattigiani’s megalopa possesses clear characters that identify it as a brachyuran megalopa larva. The immature status of the specimen is demonstrated by its small overall size, the immature appearance of the antennules and antennae, and the small pleon extending behind (rather than folded beneath) the cephalothorax. The absence of exopods, absence of a forked telson, large eyes, and wide carapace argue strongly against a zoea stage, as does the overall habitus. The positioning and bending of thoracopods 5–8, especially the angle of the last two legs on the specimen’s left side (right side in Fig. 2a ), are very characteristic of other extant brachyuran megalopa larvae (compare Fig. 2g and Fig. 5a,b ). Some common megalopal characters are not seen in Frattigiani’s megalopa, most obvious of which are the serrate, recurved setae (presumed to be sensory in nature) that are typical of the dactylus of thoracopod 8 (=pereopod 5, the last walking leg). However, setae in general are not preserved well in fossil crustaceans and are not seen elsewhere in Frattigiani’s megalopa; furthermore, these distinctive setae are not known from all families of extant crabs [14] . So their ‘absence’ here is not viewed by us as significant. 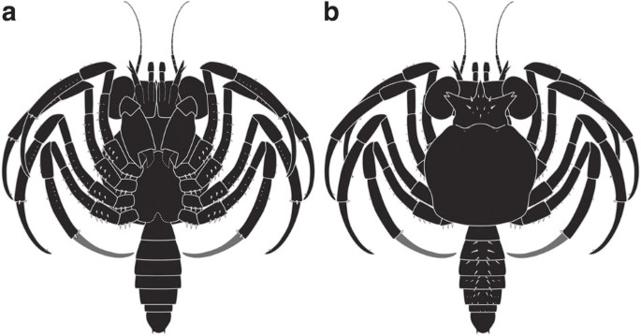Figure 5: Schematic reconstruction of Frattigiani’s megalopa. (a) Reconstruction of ventral aspects; exact outline of movable finger of chela unclear, therefore the line is stippled. Also the more proximal parts of antennula and antenna are stippled for the same reason. Sternum morphology also unclear (only indicated by the surrounding appendages), drawn similar to modern forms. (b) Reconstruction of dorsal aspects. Exact morphology of last thoracopod unclear, here drawn sub-similar to more anterior ones. Figure 5: Schematic reconstruction of Frattigiani’s megalopa. ( a ) Reconstruction of ventral aspects; exact outline of movable finger of chela unclear, therefore the line is stippled. Also the more proximal parts of antennula and antenna are stippled for the same reason. Sternum morphology also unclear (only indicated by the surrounding appendages), drawn similar to modern forms. ( b ) Reconstruction of dorsal aspects. Exact morphology of last thoracopod unclear, here drawn sub-similar to more anterior ones. Full size image Anomuran decapods, although having a comparable life history that involves a series of zoeal larvae followed by a single megalopa stage, differ from brachyurans in details of their developmental stages. The typical anomuran megalopa (often called a glaucothoe) differs significantly from that of brachyurans and from Frattigiani’s megalopa in the developmental degree of the pleon. Anomuran megalopae usually have a better-developed pleon with pronounced uropods [23] , [24] , [25] , [26] . The pleon of brachyuran megalopae is significantly more slender and is posteriorly tapering, and the uropods are inconspicuous to virtually absent [14] , [27] , [28] , [29] . The pleon of Frattigiani’s megalopa is also very slender, and uropods are not apparent. It is unlikely that the uropods became lost during the fossilisation process as the specimen is so well-preserved otherwise and because uropods indeed rarely become detached, neither in living (extant) anomuran megalopae nor in fossil adult decapods. Furthermore, the shape and position of thoracopods 5–8 is absolutely similar to that seen in modern crab megalopae, with a distinctive folding between articles 4 and 5 (merus and carpus) [14] . Such a position also appears occasionally in, but is not truly typical of, extant anomuran megalopae [26] . Frattigiani’s megalopa provides a minimum age for the evolution of the true crab (brachyuran) megalopa. In comparison to supposed ‘primitive’ megalopa larvae of dromiids or homolids (e.g., ref. 14 , Fig. 8A–I), Frattigiani’s megalopa appears quite ‘modern’ (compare to Fig. 2g ) There is virtually nothing present in the fossil specimen that would exclude, for example, an alliance of this fossil with megalopae of Panopeidae, Xanthidae, Sesarmidae, or Varunidae (ref. 14 , Figs 9Q, 9V, 10A, and 10B, respectively). Certain extant groups have features that could be used to exclude a possible relationship: the width of the megalopal carapace in Pinnotheridae, for example (ref. 14 , Fig. 10G, H), or the absence of strong sternal spines seen in some representatives of Portunidae (e.g., ref. 14 , Fig. 9T). But overall, Frattigiani’s megalopa could easily pass for the larva of an extant group. There are close to 180 higher taxonomic groups (families) of extant brachyuran crabs, yet full larval descriptions are known from very few of them [14] , making it impossible to more accurately assign Frattigiani’s megalopa to any of these groups with certainty. Thus, although crabs were only beginning to undergo their rapid radiation in the late Jurassic, not only their adult morphotype but also the specific morphology of the megalopa larvae appears to have been already established. Although we can only speculate about the morphology of the earlier ontogenetic stages (the zoea larvae of the Jurassic forms), the morphology of the megalopa indicates that the life-history strategy of modern brachyurans had already evolved. This pattern is quite different from those seen in lineages of lobsters. Here the larval stages of early representatives are often significantly less specialised than those of modern forms [17] , [18] , [19] . It is furthermore interesting to note that apparently the niche-differentiation between larvae and adults, often thought to be an important factor for evolutionary success, also appears to have already evolved, even though the true success of crabs would not be achieved for some tens of millions of years later. The comparably modern morphology of Frattigiani’s megalopa could be interpreted in two ways. One possibility is that, in addition to the morphologically ‘primitive’ prosopidans and other crabs known from the Jurassic, it is possible that other, more derived, brachyuran crabs also had evolved by the late Jurassic and are simply not represented well in the fossil record as adults. The second interpretation is that the morphology of the megalopa stage of these ancient crabs was already ‘modern,’ which could also mean that the supposed ancestral megalopa morphologies like those of dromiids, homolids and latreillids are in fact more derived than we thought. Case 1 seems rather unlikely, as the adults would have a significantly higher preservation potential than the larvae. In other decapod groups, reconstructions of ancestral developmental patterns, or larval forms, which are based exclusively on modern forms may lead to quite different results, compared to cases in which fossil evidence is taken into account [17] , [18] . This demonstrates that developmental patterns and larval forms can become specialised in various lineages and obscure the true ancestral pattern. Therefore, we see it as more likely that the morphology of Frattigiani’s megalopa, although appearing relatively modern, represents a comparably ancestral morphology. A precise character evolution will have to await a phylogenetic analysis including fossil evidence and developmental data, but also a re-evaluation of fossil material in a strict comparative approach. As has been demonstrated, information from the megalopa stage has the potential to provide phylogenetically important data [30] , [31] . Despite these challenges, the new fossil provides a hint that we will need to re-consider certain aspects of brachyuran evolution. Modern brachyuran megalopae, where known, are mostly ‘opportunistic’ feeders, usually predators or scavengers, as are many adult crabs [14] . They are known to feed on other zooplankton, other crustaceans, and small fish. As the ventral morphology of the fossil species is so similar to modern forms, we can surmise that is was also a planktic predator and scavenger of comparably small size. There are stomatopod larvae of comparable size known from the lithographic limestones of southern Germany [32] , but most of their appendages are unknown, and it is unclear whether these stages were already predatory, as certain early stages of stomatopods still lack the raptorial apparatus [33] . Thus, the megalopa larva described here provides new insights into the early evolution of crabs, but it also allows some insight into the late Jurassic ecosystem; it is our first definite evidence for this specific ecological guild in the fauna of the lithographic limestones. The find also shows the preservational capabilities of this Mesozoic ecosystem and indicates that more exceptional finds should appear in the future. Origin of specimens The single specimen was found in the Solnhofen Lithographic Limestones (close to Blumenberg) by Roger Frattigiani (September 2013) and is now part of the collections of the Staatliches Museum für Naturkunde Stuttgart (SMNS 70265). Documentation The specimen was documented by composite-fluorescence imaging (workflow in refs 34 , 35 , 36 ) on a Keyence BZ-9000 fluorescence microscope. Additionally, photographs were taken under cross-polarised light with a Canon EOS Rebel T3i camera and a MP-E 65 mm macro lens. Light was provided by a Canon Macro Twin Lite MT-24EX Flash or a MeiKe LED Macro Ring Flash FC 100. In addition to a composite image, a stereo image and virtual surface reconstructions, based on stacks in two different magnifications, were recorded [37] , [38] . For the schematic reconstruction of the specimen ( Fig. 5 ), dorsal and ventral aspects of the specimen were separated ‘by hand’ on the high-resolution images. How to cite this article: Haug, J. T. et al . A 150-million-year-old crab larva and its implications for the early rise of brachyuran crabs. Nat. Commun . 6:6417 doi: 10.1038/ncomms7417 (2015).